Transmembrane insertion of twin-arginine signal peptides is driven by TatC and regulated by TatB The twin-arginine translocation (Tat) pathway of bacteria and plant chloroplasts mediates the transmembrane transport of folded proteins, which harbour signal sequences with a conserved twin-arginine motif. Many Tat translocases comprise the three membrane proteins TatA, TatB and TatC. TatC was previously shown to be involved in recognizing twin-arginine signal peptides. Here we show that beyond recognition, TatC mediates the transmembrane insertion of a twin-arginine signal sequence, thereby translocating the signal sequence cleavage site across the bilayer. In the absence of TatB, this can lead to the removal of the signal sequence even from a translocation-incompetent substrate. Hence interaction of twin-arginine signal peptides with TatB counteracts their premature cleavage uncoupled from translocation. This capacity of TatB is not shared by the homologous TatA protein. Collectively our results suggest that TatC is an insertase for twin-arginine signal peptides and that translocation-proficient signal sequence recognition requires the concerted action of TatC and TatB. Twin-arginine (Tat)-specific protein translocation machineries are found in bacteria, archaea and plant chloroplasts. Tat machineries have the remarkable property to transport fully folded proteins across cellular membranes. These proteins are specifically directed to the Tat pathway by signal peptides harbouring a conserved S- R - R -x-F-L-K sequence motif (RR-signal peptides). The current knowledge on the Tat pathway has comprehensively been reviewed [1] , [2] , [3] , [4] , [5] . In Gram-negative bacteria and plant chloroplasts, Tat machineries are composed of three membrane proteins that in bacteria are termed TatA, TatB and TatC. TatA encompasses a single transmembrane domain and a cytosolically located amphipathic helix [6] , [7] that is followed by an unstructured C-terminus. Despite contradictory reports in the past [8] , [9] , [10] , recent reports confirm an N out -orientation of the transmembrane helix of TatA [11] , [12] . The homologous, yet functionally distinct TatB subunit has the same predicted structure as TatA. TatC on the other hand, possesses six predicted transmembrane helices with the N- and C-termini of the protein facing the cytoplasm. In E. coli , TatA is expressed at about 25- and 50-fold higher levels than TatB and TatC, respectively, but might be much less abundant in plant chloroplasts [13] . Two main complexes made up of the three Tat subunits have been described in E. coli : a 360–700 kDa complex that is composed of oligomers of a 1:1 TatB/TatC core unit with varying amounts of TatA associated [14] , [15] , and an oligomeric TatA complex consisting of varying numbers of TatA protomers (100–700 kDa) [15] , [16] , [17] , [18] . The TatBC complex is involved in binding RR-signal peptides as shown by multiple experimental strategies, such as (1) interference of precursor binding to the Tat translocase by antibodies directed against TatB and TatC [19] , (2) comigration of precursor with a TatBC complex on Blue-native-polyacrylamide gel electrophoresis (PAGE) [20] , (3) copurification of precursor, TatB and TatC upon membrane solubilization [16] , [21] , (4) chemical and site-directed cross-linking [22] , [23] , [24] and (5) identification of TatBC suppressor mutations of export-defective Tat signal peptides [25] , [26] . The identification of binding sites both on TatBC, as well as on RR-signal peptides has been the subject of several reports. Thus crosslinking studies have repeatedly revealed a close proximity between the consensus RR-motif and TatC [23] , [24] , [27] . These signal peptide-TatC cross-links persist even in the absence of TatB [23] pointing towards TatC as the primary recognition site for RR-signal sequences. Consistent with this notion, fusions between RR-signal peptides and PhoA were found to be redirected to the Sec translocon, if TatC was missing [28] . Using site-specific photo crosslinking the signal peptide-binding site of TatC was recently mapped to its cytosolic N-terminus and first cytosolic loop [29] . In full agreement with these crosslinking studies, suppressor mutations in TatC that partially alleviate the transport block of KQ- and KK-mutant precursors map exactly to the same two domains of TatC [25] , [30] . Thus TatC provides a superficially exposed precursor recognition site. The homooligomeric TatA complex forms pore-like structures [31] , in which the transmembrane helices of TatA are arranged as rings [32] . These findings gave rise to a current model, according to which the TatA complexes represent individually form-fitting transmembrane conduits for folded Tat substrates. In this model, an RR-precursor following its binding to the TatBC complex would initiate the customized recruitment of TatA, a process that also requires the proton-motive force (PMF). Whether TatA is recruited only from membrane-integrated TatA protomers or also from a soluble pool of TatA is still an issue [33] . Despite these insights there are a number of unsettled issues. Thus, some Tat-directed substrates might interact with the membrane bilayer before binding to TatBC [34] , [35] , [36] . Furthermore, Tat transport was shown to proceed even in conditions, in which the Tat(A)BC and TatA complexes mentioned above could not be recovered to detectable levels, casting some doubt on those two complexes being true correlates of functional events during Tat-dependent transport [37] . Similarly, enterobacteria contain an additional paralog of TatA, called TatE, that can functionally replace TatA although it forms much smaller complexes than TatA [38] . According to the above model, TatA and TatB are predicted to fulfill quite diverse functions. In fact, single tatA and tatB knockout mutants of E. coli both show a tat phenotype despite a 20% sequence identity between both proteins. On the contrary, many Gram-positive bacteria naturally express only TatA and TatC orthologues. This suggests that in these organisms TatA has the functional roles of both TatA and TatB, which indeed could be verified experimentally [39] . Consistent with natural bifunctional TatA proteins, TatA variants that were altered at their extreme N-termini have been isolated that are able to suppress a TatB deficiency in E. coli [40] . Here we experimentally exploited a TatB deficiency to unravel the unanticipated ability of TatC to act as a membrane insertase of Tat signal peptides. Correct cleavage of RR-precursors in the absence of TatB Using the model Tat substrate TorA-MalE, distinct N-terminal mutations in tatA were previously isolated, that are able to suppress a complete lack of TatB in E. coli cells. These mutations render TatA a bifunctional TatA/B component [37] , [40] , much like in Gram-positive bacteria that naturally do not express a TatB subunit [41] . We were unable to detect the suppressing phenotype of those tatA variants in vitro , probably because of the rather low overall translocation efficiency of our cell-free system. When performing these experiments we, however, noticed that E. coli membrane vesicles harbouring only TatC and TatA nevertheless led to a proteolytic processing of the TorA-MalE precursor. This is shown in Fig. 1a that depicts the radiolabelled precursor TorA-MalE335 after in vitro synthesis in the absence or presence of TatABC- and TatAC-containing membrane vesicles. MalE is the periplasmic maltose-binding protein of E. coli, which naturally is exported through the Sec translocon but can be directed to the Tat system, if its Sec signal sequence is replaced by the RR-signal of the Tat substrate TMAO reductase (TorA) [42] . Here we used the fusion protein TorA-MalE335 containing a C-terminally truncated MalE-moiety that lacks the inherent protease resistance of full-size MalE thereby allowing us to monitor its transport into membrane vesicles via protease protection. Thus TorA-MalE335 when synthesized by in vitro transcription/translation was completely digested by externally added proteinase K (PK; Fig. 1a , compare lanes 1 and 2). Following synthesis in the presence of inside-out inner membrane vesicles (INV) prepared from a TatABCD-overproducing E. coli strain (Tat + -INV), a significant amount of TorA-MalE335 was processed to a smaller species (lane 3). The processing product was resistant to PK (lane 4) suggesting that it had been translocated into the lumen of the vesicles and that it originated from cleavage by the vesicle-borne signal peptidase (leader peptidase). As usually observed for INV [43] , translocation was not strictly coupled to cleavage, because some of the precursor of TorA-MalE335 was also found to be PK-resistant (lane 4). This material was, however, slightly shorter than the non PK-treated precursor (compare lanes 3 and 4; see also figures below). We assume that this shift in molecular mass was due to a PK-mediated removal a few N-terminal amino acids preceding the RR-consensus motif from the otherwise membrane-protected TorA-signal peptide. 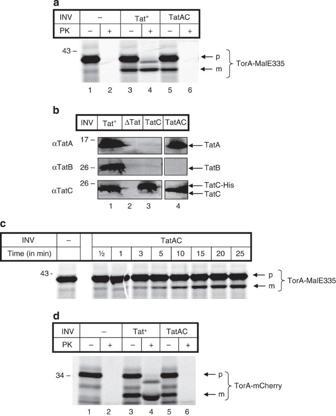Figure 1: Twin-arginine precursors are proteolytically processed in the absence of TatB. (a) The radiolabelled precursor TorA-MalE335 was synthesizedin vitroby coupled transcription/translation in the absence or presence of TatABC- and TatAC-containing inside-out INV. Samples were digested with PK to visualize protease-resistant, that is, translocated, precursor (p) and mature (m) form of TorA-MalE335. Samples were separated by SDS–PAGE and visualized by phosphorimaging. Tat+-INV prepared from a TatABCD-overproducingE. colistrain show processing of the precursor of TorA-MalE335 and render its mature part and some precursor of slightly reduced size resistant to PK. In contrast, TatAC-INV prepared from a TatAC-overproducing Δtat E. colistrain lacking TatB show a complete block in translocation, as no PK-resistant material was obtained. Nevertheless, these TatAC-INV proteolytically process TorA-MalE335 generating a fragment of the same electrophoretic mobility that mature TorA-MalE335 displays after its translocation into the Tat+-INVs. (b) The indicated vesicles were dissolved in SDS–PAGE loading buffer and the Tat components were separated by SDS–PAGE and visualized by western blotting using polyclonal antibodies against TatA, TatB or TatC. Note that TatC-INV were prepared from a Δtatstrain expressing a His-tagged version of TatC. (c) TorA-MalE335 was synthesized for 10 min. TatAC-INV were added and incubations stopped at the indicated times by adding TCA. Cleavage of TorA-MalE in the absence of TatB thus turned out to be a time-dependent process. (d) As in (a) using the Tat model precursor TorA-mCherry. As observed for TorA-MalE, the TatB-lacking TatAC-INV are not able to translocate TorA-mCherry, although they cause its proteolytic processing. Figure 1: Twin-arginine precursors are proteolytically processed in the absence of TatB. ( a ) The radiolabelled precursor TorA-MalE335 was synthesized in vitro by coupled transcription/translation in the absence or presence of TatABC- and TatAC-containing inside-out INV. Samples were digested with PK to visualize protease-resistant, that is, translocated, precursor (p) and mature (m) form of TorA-MalE335. Samples were separated by SDS–PAGE and visualized by phosphorimaging. Tat + -INV prepared from a TatABCD-overproducing E. coli strain show processing of the precursor of TorA-MalE335 and render its mature part and some precursor of slightly reduced size resistant to PK. In contrast, TatAC-INV prepared from a TatAC-overproducing Δ tat E. coli strain lacking TatB show a complete block in translocation, as no PK-resistant material was obtained. Nevertheless, these TatAC-INV proteolytically process TorA-MalE335 generating a fragment of the same electrophoretic mobility that mature TorA-MalE335 displays after its translocation into the Tat + -INVs. ( b ) The indicated vesicles were dissolved in SDS–PAGE loading buffer and the Tat components were separated by SDS–PAGE and visualized by western blotting using polyclonal antibodies against TatA, TatB or TatC. Note that TatC-INV were prepared from a Δ tat strain expressing a His-tagged version of TatC. ( c ) TorA-MalE335 was synthesized for 10 min. TatAC-INV were added and incubations stopped at the indicated times by adding TCA. Cleavage of TorA-MalE in the absence of TatB thus turned out to be a time-dependent process. ( d ) As in ( a ) using the Tat model precursor TorA-mCherry. As observed for TorA-MalE, the TatB-lacking TatAC-INV are not able to translocate TorA-mCherry, although they cause its proteolytic processing. Full size image When instead INV were used that had been prepared from a strain only expressing TatA and TatC ( Fig. 1b , lane 4) no PK-resistant material was obtained ( Fig. 1a , lane 6), confirming a complete block in translocation when the TatB component was missing. Despite their translocation deficiency, these vesicles led to a substantial proteolytic processing of TorA-MalE335 ( Fig. 1a , lane 5). Cleavage of TorA-MalE335 by TatAC-INV was a time-dependent process ( Fig. 1c ) and was not a unique feature of this precursor, but was similarly obtained for the Tat model protein TorA-mCherry ( Fig. 1d , lane 5) and TorA-PhoA (see below Fig. 2c ). 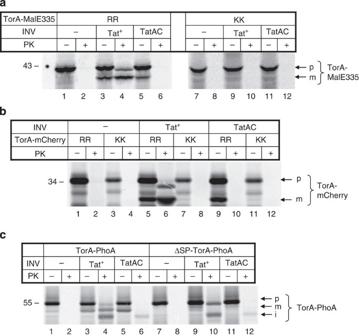Figure 2: RR-motif and cleavage site mutations abolish processing by TatB-deficient TatAC-vesicles. (a,b)In vitrosynthesis of the radiolabelled TorA-MalE335 and TorA-mCherry precursors in the absence and presence of INV containing TatABC (Tat+) or TatAC. Transport and processing by Tat+-INV are completely abolished if the signal sequences of both precursors carry the KK-mutation. Similarly, cleavage of the TorA-precursors by the TatB-deficient TatAC-vesicles does not occur when the authentic RR-motif is mutated to KK. (c) As in (a,b) comparing the RR-precursor TorA-PhoA to its non-cleavable variant ΔSP-TorA-PhoA. As expected, the processed mature form of wild-type TorA-PhoA recovererd from Tat+-INV after PK-treatment (m) is not obtained for ΔSP-TorA-PhoA (compare lanes 4 and 10). Furthermore, no processed form of the ΔSP-TorA-PhoA precursor is detectable in TatB-deficient TatAC-vesicles (compare lanes 5 and 11), indicating that cleavage requires an intact signal peptidase cleavage site. The band labelled (i) is a translocation intermediate uniquely observed for TorA-PhoA27. Figure 2: RR-motif and cleavage site mutations abolish processing by TatB-deficient TatAC-vesicles. ( a , b ) In vitro synthesis of the radiolabelled TorA-MalE335 and TorA-mCherry precursors in the absence and presence of INV containing TatABC (Tat + ) or TatAC. Transport and processing by Tat + -INV are completely abolished if the signal sequences of both precursors carry the KK-mutation. Similarly, cleavage of the TorA-precursors by the TatB-deficient TatAC-vesicles does not occur when the authentic RR-motif is mutated to KK. ( c ) As in ( a , b ) comparing the RR-precursor TorA-PhoA to its non-cleavable variant ΔSP-TorA-PhoA. As expected, the processed mature form of wild-type TorA-PhoA recovererd from Tat + -INV after PK-treatment (m) is not obtained for ΔSP-TorA-PhoA (compare lanes 4 and 10). Furthermore, no processed form of the ΔSP-TorA-PhoA precursor is detectable in TatB-deficient TatAC-vesicles (compare lanes 5 and 11), indicating that cleavage requires an intact signal peptidase cleavage site. The band labelled (i) is a translocation intermediate uniquely observed for TorA-PhoA [27] . Full size image Processing of the TorA-precursors by the TatB-deficient TatAC-vesicles required an intact RR-consensus motif ( Fig. 2a ). Replacement of the essential RR-residues of the TorA-MalE335 and TorA-mCherry fusion proteins by pairs of lysines resulted in the expected block of translocation and processing of both precursors by TatABC-containing membrane vesicles ( Fig. 2a , compare lanes 3, 4 to 9, 10; Fig. 2b , lanes 5–8). Importantly, processing of the KK-mutant TorA-precursors by the TatAC-vesicles lacking TatB was also totally abolished (compare in Fig. 2a , lanes 5 and 11; in Fig. 2b , lanes 9 and 11) indicating that recognition of the authentic twin-arginine motif by the TatB-deficient TatAC-vesicles was a prerequisite for them to cleave unaltered TorA-precursors. This would not be the case, if processing of the precursor were due to unspecific proteases. In order to test if processing of the TorA-precursors in the absence of TatB was in fact executed by signal peptidase, we made use of a mutant TorA-PhoA precursor, the signal peptide cleavage site of which had been inactivated by mutating its sequence from ATA-AQA to ATL-LQA [27] . This non-cleavable variant of TorA-PhoA was not processed by the TatAC-vesicles lacking TatB ( Fig. 2c , lanes 5 and 11). Thus the findings depicted in Fig. 2 suggest that despite lacking TatB, TatAC-vesicles recognize the twin-arginine motif of the TorA-signal peptide and mediate access of its cleavage site to signal peptidase. TatB prevents premature signal peptide cleavage Tat-specific transmembrane translocation requires the PMF at the membrane. Accordingly, the protonophore carbonyl cyanide m-chlorophenyl-hydrazone (CCCP) completely abolished translocation of TorA-MalE335 into TatABC-INV ( Fig. 3a , compare lanes 6 and 8). Of note, no signal sequence cleavage by TatABC-INV was observed in the presence of CCCP (compare lanes 5 and 7), indicating that the wild-type Tat translocase allows processing of TorA-MalE335 only in conjunction with translocation. On the contrary, signal sequence cleavage obtained by the TatAC-vesicles in the absence of TatB was virtually unaffected by CCCP (compare lanes 9 and 11). Hence in this experimental setup, translocation of the twin-arginine signal peptide per se , as opposed to that of the complete precursor protein, proceeds without PMF. 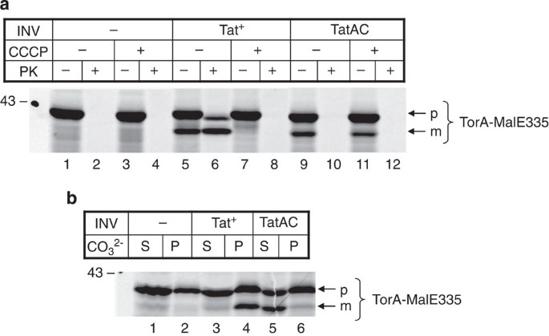Figure 3: TorA-signal sequence cleavage is independent of PMF in the absence of TatB. (a) TorA-MalE335 was synthesized in the absence or presence of the indicated vesicles, one part each containing the uncoupler CCCP at 0.1 mM, the other only the solvent dimethylsulphoxide. Whereas CCCP completely blocks translocation of TorA-MalE335 into Tat+-INV (lane 8) and thereby also prevents processing by the signal peptidase (lane 7), processing obtained by the TatB-lacking vesicles is unaffected by adding CCCP (lane 11). Thus, premature processing of TorA-MalE335 uncoupled from translocation of its MalE-moiety obviously results from a PMF-independent translocation of the TorA signal sequence cleavage site across the membrane. (b) After synthesis of TorA-MalE335 without or with the indicated INV, samples were treated with 0.2 M Na2CO3. Most of the processed form of TorA-MalE335 obtained from Tat+-INV is carbonate-resistant due to translocation into the vesicles and, therefore, sediments with the INV (P, pellet). In contrast, TorA-MalE335 processed by TatAC-INV but not translocated because of a lack of TatB is released into the carbonate-soluble fraction (S, supernatant). Figure 3: TorA-signal sequence cleavage is independent of PMF in the absence of TatB. ( a ) TorA-MalE335 was synthesized in the absence or presence of the indicated vesicles, one part each containing the uncoupler CCCP at 0.1 mM, the other only the solvent dimethylsulphoxide. Whereas CCCP completely blocks translocation of TorA-MalE335 into Tat + -INV (lane 8) and thereby also prevents processing by the signal peptidase (lane 7), processing obtained by the TatB-lacking vesicles is unaffected by adding CCCP (lane 11). Thus, premature processing of TorA-MalE335 uncoupled from translocation of its MalE-moiety obviously results from a PMF-independent translocation of the TorA signal sequence cleavage site across the membrane. ( b ) After synthesis of TorA-MalE335 without or with the indicated INV, samples were treated with 0.2 M Na 2 CO 3 . Most of the processed form of TorA-MalE335 obtained from Tat + -INV is carbonate-resistant due to translocation into the vesicles and, therefore, sediments with the INV (P, pellet). In contrast, TorA-MalE335 processed by TatAC-INV but not translocated because of a lack of TatB is released into the carbonate-soluble fraction (S, supernatant). Full size image Processing of the signal peptide, with the mature part of TorA-MalE335 remaining untranslocated, invokes a hairpin-like insertion of the signal sequence and early mature part of TorA-MalE335 into the membrane of TatAC-vesicles. Consistent with such a scenario, the signal sequence-less MalE-moiety when deprived of its membrane anchor by the processing activity of the TatAC-vesicles could largely be extracted by sodium carbonate ( Fig. 3b , lanes 5 and 6). This was in contrast to the processed form of TorA-MalE335 obtained from TatABC- (Tat + -) INV (lanes 3 and 4), in which case translocation of the MalE-moiety rendered it for the most part carbonate-resistant. Moreover, these findings suggest that in the presence of an intact TatABC translocase, a futile cleavage of the twin-arginine signal peptide uncoupled from translocation of the passenger protein is prevented by the presence of TatB. This property seems to be unique for TatB as it was not shared by TatA being present in comparable amounts in TatAC- and TatABC-vesicles ( Fig. 1b ). TatC mediates membrane insertion of an RR-signal sequence Next we prepared INV from an E. coli strain that expressed TatC as the only Tat component ( Fig. 1b , lane 3). Clearly these TatC-INV allowed undiminished processing of TorA-mCherry and TorA-MalE335 when compared with TatAC-vesicles ( Fig. 4a , compare lanes 5 and 7). That signal sequence cleavage by TatC-only INV was in fact promoted by TatC, was demonstrated by a direct comparison between TatC-INV and those prepared from a total tat deletion strain. Although these ΔTat vesicles gave rise to some degradation products of both precursors (and all others tested), none of these fragments comigrated with the signal sequence-less mature forms processed by the TatAC- and TatC-INV (compare lanes 5 and 7 to 9). These results would be consistent with TatC functioning as an insertase of a twin-arginine signal peptide thereby mediating its exposure to signal peptidase ( Fig. 4b , left). 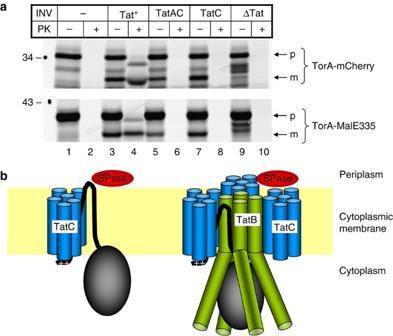Figure 4: TatC alone can translocate TorA-precursor signal sequence cleavage sites. (a) TorA-mCherry and TorA-MalE335 were synthesized in the absence and presence of the indicated vesicles. TatC-INV were prepared from a Δtatstrain expressing only TatC, while ΔTat-INV do not contain any Tat component. Vesicles containing only TatC allow the same processing of TorA-mCherry and TorA-MalE335 as TatAC-INV. As expected, correct signal sequence cleavage is, however, not observed for vesicles prepared from a totaltatdeletion strain. The reason for the partial instability of both precursors in the presence of ΔTat-INV is not clear. (b) Model of possible TatC/TatB-signal sequence interactions. The yellow bar represents the lipid bilayer. The TatC molecule is depicted by six transmembrane helices (blue). Four TatB monomers are shown (green cylinders) following a recent report45. TatB and TatC form 1:1 complexes14. For clarity, the front TatC molecule has been omitted. The twin-arginine signal sequence (++) is represented by a black line and the folded mature part of a RR-precursor by a black ellipse. TatC acts as an insertase of a twin-arginine signal peptide thereby mediating its exposure to signal peptidase (SPase). Embedding the signal sequence in a TatBC-binding pocket interferes with a premature cleavage by signal peptidase. Figure 4: TatC alone can translocate TorA-precursor signal sequence cleavage sites. ( a ) TorA-mCherry and TorA-MalE335 were synthesized in the absence and presence of the indicated vesicles. TatC-INV were prepared from a Δ tat strain expressing only TatC, while ΔTat-INV do not contain any Tat component. Vesicles containing only TatC allow the same processing of TorA-mCherry and TorA-MalE335 as TatAC-INV. As expected, correct signal sequence cleavage is, however, not observed for vesicles prepared from a total tat deletion strain. The reason for the partial instability of both precursors in the presence of ΔTat-INV is not clear. ( b ) Model of possible TatC/TatB-signal sequence interactions. The yellow bar represents the lipid bilayer. The TatC molecule is depicted by six transmembrane helices (blue). Four TatB monomers are shown (green cylinders) following a recent report [45] . TatB and TatC form 1:1 complexes [14] . For clarity, the front TatC molecule has been omitted. The twin-arginine signal sequence (++) is represented by a black line and the folded mature part of a RR-precursor by a black ellipse. TatC acts as an insertase of a twin-arginine signal peptide thereby mediating its exposure to signal peptidase (SPase). Embedding the signal sequence in a TatBC-binding pocket interferes with a premature cleavage by signal peptidase. Full size image Structural requirements for premature cleavage The situation depicted in Fig. 4b (left) requires that both the signal sequence preceding the cleavage site and the early mature region of the precursor allow the loop to extend onto signal peptidase. To prove this, we also employed the two natural E. coli Tat substrates SufI (FtsP) and AmiC. As shown in Fig. 5a , although both in vitro synthesized precursors were translocated into and concomitantly cleaved by TatABC-INV (lanes 3 and 4), no proteolytic processing was obtained by TatAC-INV lacking TatB (lane 5), which is in clear contrast to the TorA-precursors described above. This result definitely rules out the possibility that cleavage of the TorA-precursors by the TatAC-INV was due to any contamination by right-side out vesicles exposing signal peptidase on their outside. Assuming that the lack of processing of pSufI and pAmiC by TatAC-vesicles originated from the nature of the signal peptides of these two RR-precursors, we replaced the authentic signal sequence of SufI by that of TorA, creating a TorA-SufI fusion protein. 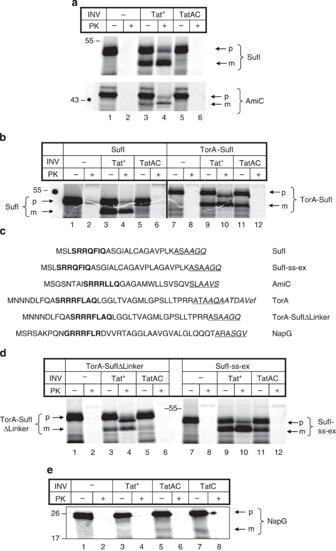Figure 5: Premature processing in the absence of TatB depends on structural determinants of RR-precursors. (a) SufI and AmiC were synthesized in the absence and presence of Tat+-INV and TatAC-INV. Both precursors are translocated into and processed by the Tat+-INV, but in contrast to TorA-precursors, are not processed by TatAC-INV lacking TatB. (b) To create the TorA-SufI fusion protein, the authentic signal sequence of SufI was replaced by that of TorA. TorA-SufI is as efficiently processed by and translocated into functional TatABC-INV as is pSufI. However, only TorA-SufI is processed by TatAC-INV lacking TatB. (c) Comparison of the different Tat signal sequences used. The consensus motifs are printed in bold letters and the six amino flanking each cleavage site are underlined. Residues of the early mature regions of each precursor are given in italic letters. The TorA signal sequence was fused to the various passenger proteins via a 10 amino acid long linker that consists of eight residues derived from mature TorA (italic capital letters) and two amino acids encoded by nucleotides that had been introduced for cloning reasons (italic lower case letters). In TorA-SufIΔLinker, this linker region was removed now connecting the first residues of SufI (AGQ) directly to the TorA signal sequence. To obtain more efficient processing, the C-terminal ATA-residues of the TorA signal peptide were changed to the SufI-derived ASA-motif. (d) To define the features that render the TorA signal sequence cleavable in the presence of TatC, the linker downstream of the cleavage site was removed from the TorA-SufI construct (TorA-SufIΔLinker) and the signal sequence of SufI was extended by six amino acids (SufI-ss-ex, cf. (c)). Compared with TorA-SufI, TorA-SufIΔLinker is less efficiently processed by the TatB-lacking TatAC- and TatC-INV, whereas compared with SufI, SufI-ss-ex acquired the capability of being processed. (e) NapG is anE. coliRR-precursor whose FeS-cofactor is not incorporated by ourin vitrosystem.In vitrosynthesized NapG, therefore, is neither processed nor translocated by Tat+-INV. Despite being translocation-incompetent, the NapG precursor is processed by the TatB-lacking TatAC- and TatC-INV yielding a cleavage product of the size of the signal sequence-less mature NapG. Figure 5b illustrates that this TorA-SufI model protein was as efficiently processed by, and translocated into functional TatABC-INV as wild-type pSufI (compare lanes 3, 4 and 9, 10). However, only TorA-SufI was processed by TatAC-vesicles (compare lanes 5 and 11). Hence, TatC-mediated transport and processing observed in the absence of TatB became manifest only for the TorA-signal peptide. Figure 5: Premature processing in the absence of TatB depends on structural determinants of RR-precursors. ( a ) SufI and AmiC were synthesized in the absence and presence of Tat + -INV and TatAC-INV. Both precursors are translocated into and processed by the Tat + -INV, but in contrast to TorA-precursors, are not processed by TatAC-INV lacking TatB. ( b ) To create the TorA-SufI fusion protein, the authentic signal sequence of SufI was replaced by that of TorA. TorA-SufI is as efficiently processed by and translocated into functional TatABC-INV as is pSufI. However, only TorA-SufI is processed by TatAC-INV lacking TatB. ( c ) Comparison of the different Tat signal sequences used. The consensus motifs are printed in bold letters and the six amino flanking each cleavage site are underlined. Residues of the early mature regions of each precursor are given in italic letters. The TorA signal sequence was fused to the various passenger proteins via a 10 amino acid long linker that consists of eight residues derived from mature TorA (italic capital letters) and two amino acids encoded by nucleotides that had been introduced for cloning reasons (italic lower case letters). In TorA-SufIΔLinker, this linker region was removed now connecting the first residues of SufI (AGQ) directly to the TorA signal sequence. To obtain more efficient processing, the C-terminal ATA-residues of the TorA signal peptide were changed to the SufI-derived ASA-motif. ( d ) To define the features that render the TorA signal sequence cleavable in the presence of TatC, the linker downstream of the cleavage site was removed from the TorA-SufI construct (TorA-SufIΔLinker) and the signal sequence of SufI was extended by six amino acids (SufI-ss-ex, cf. ( c )). Compared with TorA-SufI, TorA-SufIΔLinker is less efficiently processed by the TatB-lacking TatAC- and TatC-INV, whereas compared with SufI, SufI-ss-ex acquired the capability of being processed. ( e ) NapG is an E. coli RR-precursor whose FeS-cofactor is not incorporated by our in vitro system. In vitro synthesized NapG, therefore, is neither processed nor translocated by Tat + -INV. Despite being translocation-incompetent, the NapG precursor is processed by the TatB-lacking TatAC- and TatC-INV yielding a cleavage product of the size of the signal sequence-less mature NapG. Full size image Figure 5c compares the signal sequence of TorA with those of SufI and AmiC. Evidently they differ in length, in particular in the distance between the consensus motif (in bold letters) and the cleavage site (underlined). In addition, all TorA-fusions so far used contain a linker sequence engineered between the TorA-signal sequence and the respective passenger protein. It was, therefore, conceivable that in the case of the TorA-signal peptide, both the comparably long hydrophobic sequence upstream of the cleavage site and the downstream linker sequence would facilitate exposure to signal peptidase. We, therefore, removed the linker from the TorA-SufI fusion. The resulting construct ( Fig. 5c , TorA-SufIΔLinker) was efficiently cleaved by, and translocated into, Tat + -INV ( Fig. 5d , lanes 3, 4) but was only poorly processed by the TatB-lacking vesicles (compare lanes 3 and 5) suggesting that the presence of the linker sequence in fact facilitates access to signal peptidase. In order to separately examine the influence of the distance between the RR-consensus motif and the cleavage site of signal peptides on the processing by the TatB-lacking vesicles, we also extended the signal sequence of SufI by duplicating the amino acid stretch AGAVPL thus generating the longer precursor SufI-ss-ex ( Fig. 5c ). Exactly as anticipated, this extension now rendered the signal sequence of SufI a much better substrate of the signal peptidase in the absence of TatB (compare Fig. 5d , lane 11 with Fig. 5b , lane 5). In addition, we also tested the natural Tat substrate NapG for processing by TatB-deficient vesicles. The signal sequence of NapG exhibits about the same overall length and distance between consensus motif and cleavage site as that of TorA ( Fig. 5c ). NapG is a FeS-containing periplasmic protein [44] . Owing to the incapability of our cell-free system to incorporate FeS-clusters, the in vitro synthesized NapG was neither processed nor translocated by Tat + -INV ( Fig. 5e , compare lanes 1,2 with 3,4). However, despite being a translocation-incompetent RR-precursor, a cleavage product of pNapG was formed by the TatB-lacking TatAC- and TatC-only vesicles (lanes 5 and 7, mNapG), that by size corresponds to the 20.5 kDa signal sequence-less form of NapG. Finally, we investigated if TatC could also in vivo be shown to mediate access of RR-precursors to the signal peptidase. For this purpose, we compared wild-type E. coli BL21(DE3) cells expressing TatC together with TatAB from the chromosomal tat operon ( Fig. 6a , TatABC-cells, lane 3) with an isogenic ΔTat derivative (lane 4) and with the ΔTat mutant uniquely expressing TatC from an arabinose-inducible plasmid-borne tatC gene (TatC-cells, lanes 1 and 2). These three strains were each transformed with plasmids encoding one of the RR-precursors pSufI, pNapG or TorA-mCherry. Cells were grown in minimal media, induced for the synthesis of the respective RR-precursor and labelled with 35 [S]-methionine/cysteine. As expected, the precursor of SufI was found processed by TatABC-cells suggesting its export to the periplasm, but remained uncleaved in ΔTat-cells, because the lack of TatABC prevented any Tat-specific translocation ( Fig. 6b , upper panel, lanes 1, 2). In agreement with the results obtained in vitro ( Fig. 5a ), cells expressing only TatC did not allow cleavage of the signal sequence of pSufI ( Fig. 6b , upper panel, lane 3). 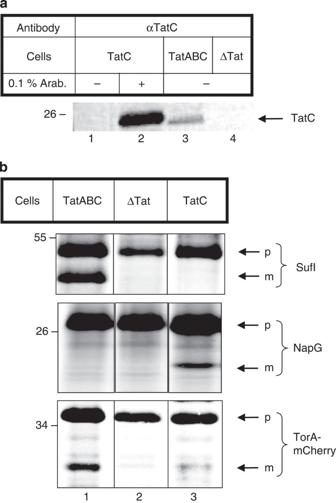Figure 6: TatC-mediated cleavage of RR-signal peptides is also observedin vivo. (a)E. coliBL21(DE3) cells used for pulse/chase labelling of RR-precursors either expressed TatC from thearaBADpromoter in the absence of TatA and TatB (TatC-cells), or TatABC from the chromosomaltatoperon (TatABC-cells), or were devoid of all Tat subunit (ΔTat-cells). Equivalent amounts of cells were blotted against anti-TatC antibodies (αTatC). (b) Cells of the indicated strains were pulse/chase-labelled as detailed in the Methods section and labelled SufI, NapG and TorA-mCherry species were purified via Ni-affinity chromatography. Note the processing of the NapG and TorA-mCherry precursors when cells expressed solely TatC. Figure 6: TatC-mediated cleavage of RR-signal peptides is also observed in vivo . ( a ) E. coli BL21(DE3) cells used for pulse/chase labelling of RR-precursors either expressed TatC from the araBAD promoter in the absence of TatA and TatB (TatC-cells), or TatABC from the chromosomal tat operon (TatABC-cells), or were devoid of all Tat subunit (ΔTat-cells). Equivalent amounts of cells were blotted against anti-TatC antibodies (αTatC). ( b ) Cells of the indicated strains were pulse/chase-labelled as detailed in the Methods section and labelled SufI, NapG and TorA-mCherry species were purified via Ni-affinity chromatography. Note the processing of the NapG and TorA-mCherry precursors when cells expressed solely TatC. Full size image In striking contrast, the same cells, which of note differ from the isogenic ΔTat-cells only by the isolated expression of TatC, allowed processing of the NapG precursor to a product of the size of mature NapG ( Fig. 6b , middle panel, lane 3). We were, however, unable to recover the same species of NapG from the TatABC-expressing cells that show processing of SufI ( Fig. 6b , lane 1). A possible explanation for this failure is that any processed, that is, translocated NapG in TatABC-containing cells is unstable when expressed in the absence of the membrane protein NapH, to which NapG is proposed to bind after transport into the periplasm [44] . Consistent with this assumption, premature cleavage of the NapG precursor by cells expressing solely TatC ( Fig. 6b , middle panel, lane 3) leads to a stable form of mature NapG protected against degradation by periplasmic proteases, because in the absence of TatA and TatB-signal sequence cleavage is uncoupled from export to the periplasm. In other words, recovery of processed NapG from cells expressing only TatC can be taken as a clue that even in vivo TatC translocates the cleavage site of appropriately sized RR-signal peptides, such as that of NapG, across the membrane. To further confirm this notion, we performed pulse-labelling also with cells expressing TorA-mCherry ( Fig. 6b , lower panel). Like pSufI, TorA-mCherry was again found processed by TatABC-cells (lane 1). Notably, the same cleavage product was formed in TatC-only cells (lane 3) again suggesting that the TatC-mediated premature cleavage of the TorA-signal peptide from this RR-precursor also occurred in vivo . In summary, our results strongly suggest that TatC is able to insert and position Tat signal sequences in a transmembrane orientation ( Fig. 4b ). Provided that the sequence context upstream and downstream of the cleavage site allows for sufficient conformational flexibility this could even lead to premature cleavage by signal peptidase, which under physiological conditions would, however, be counteracted by TatB. The experiments described here suggest that TatC, which thus far has mainly been characterized as part of a Tat-specific signal sequence receptor, additionally seems to function in the generation of the transmembrane orientation of RR-signal sequences. This signal peptide-insertase activity of TatC neither requires TatB nor TatA. As depicted in the model of Fig. 4b , TatC would thus drive a hairpin-like embedment of RR-precursor proteins in the target membrane. Under normal conditions, that is in the presence of TatB, the TatC-mediated insertion would lead to the accommodation of the Tat signal sequence in a binding pocket jointly formed by TatC and TatB. As previous studies have revealed an oligomeric assembly of TatB [21] in particular when interacting with RR-precursors [45] , we depicted in the model of Fig. 4b TatB as the tetrameric complex previously proposed following a cysteine crosslinking analysis [46] . The model further suggests that fixation of the Tat signal sequence between TatC and TatB helps to prevent an exposure of the signal sequence cleavage site to signal peptidase before translocation of the mature part of the precursor protein. This idea is derived from the findings described here that a Tat translocase lacking TatB can allow processing of a translocation-incompetent RR-precursor ( Fig. 5e , lanes 5, 7) and the premature removal of the signal sequence even from an otherwise translocation-proficient Tat substrate ( Fig. 3a , lane 11). A hairpin-like insertion of RR-precursors into TatBC would be a corollary of the N-proximal part of a Tat signal peptide being captured at the cytosolic side of the membrane. Such a precursor topology is consistent both with a superficially exposed precursor binding site provided by TatC [29] and the protease accessibility demonstrated for RR-precursors bound to the thylakoidal Tat translocase [47] , [48] . Similarly all TorA-fusions analysed in here were found to become slightly shortened by PK added after their translocation into Tat + -vesicles ( Fig. 1a , lane 4; Fig. 1d , lane 4; Fig. 2c , lane 10; Fig. 5b , lane 10). This phenomenon became manifest because membrane vesicles as used here usually fail to process all translocated precursor molecules by their resident signal peptidase. As uncleaved precursor molecules remain membrane-anchored they consequently constitute a target for externally added proteases. The presumed insertase activity of TatC would position the signal sequence and, depending on the depth of insertion, some amino acids of the early mature region of an RR-precursor into a membrane-embedded binding pocket, which the model of Fig. 4b suggests to be formed by TatC and TatB. A deep loop-like insertion of an RR-precursor between TatB and TatC is experimentally supported by (1) suppressor mutations located near the trans -sided N-terminus of TatB that compensate the translocation defect of mutant TorA-precursors [25] , [26] ; (2) crosslinking of the same area of TatB to the precursors of TorA and SufI [45] ; (3) preferential crosslinking of the hydrophobic part of Tat signal peptides located downstream of the RR-consensus motif to TatB [23] , [24] , [27] ; (4) site-specific crosslinking between transmembrane helices of TatC and TatB [49] . If TatC catalyses the transmembrane insertion of Tat signal peptides it would function in a similar way as the YidC protein insertase present in bacterial cytoplasmic membranes, which is involved in the insertion process of α-helical membrane proteins [50] . Similar to TatC, members of the YidC/Oxa1/Alb3 family, which are also found in mitochondria and chloroplasts, harbour five to six predicted transmembrane domains and are believed to form a platform for the insertion of the hydrophobic transmembrane helices of their substrates. Whereas YidC clients in general are released into the lipid bilayer after they adopted their transmembrane orientation, RR-signal peptides seem to remain attached to TatC even after translocation of the entire mature domain [24] . In summary, the model shown in Fig. 4b proposes that after recognition of the RR- consensus motif by TatC at the cytosolic surface of the Tat translocase, the proposed insertase activity of TatC inserts and accommodates the signal peptide in a concerted TatBC-binding groove, a process that most likely also involves reorientation events that might depend on the function of TatB and the presence of the PMF [47] , [51] . Recent data obtained with the E. coli Tat machinery suggest that monomeric TatA might be recruited at this early stage in a PMF-sensitive manner [52] . Before the start of translocation a single precursor molecule has been found in contact with more than one TatB molecule [45] . Whether this stage simply reflects the interaction of an RR-precursor with preformed oligomeric TatBC structures [21] , [22] , [53] or results from a precursor-mediated oligomerization of TatBC units is not known. An oligomeric TatB structure formed around a TatC-anchored precursor could then serve as the nucleation point for the recruitment of numerous TatA protomers and even the formation of higher-order oligomeric TatABC complexes eventually allowing the transmembrane passage of the precursor. Assembly of TatA on a TatB-based scaffold would allow a lateral access of the substrate to the protein-conducting structure rather than having to invoke a transfer event between a receptor complex and a pore structure. During all these assembly steps the RR-precursor would remain fixed via its signal sequence to its initial TatC-binding site. It is even conceivable that such a stable association of the Tat signal peptide with TatC is a prerequisite for forming and maintaining the Tat-specific protein conduit in the membrane. Completion of translocation, which in fact can proceed without removal of the signal sequence [24] , [54] , would then lead to cleavage of the RR-precursor by signal peptidase and a subsequent dissociation of the signal peptide from TatBC would be the trigger for the dissociation of the Tat translocase. Plasmids Plasmids were all verified by DNA sequencing. Plasmid pPJ7 (pET22b+/NapG) was constructed by PCR using total DNA of E. coli Top10 cells as template and the primers 5-NapG NdeI and 3-NapG XhoI ( Supplementary Table S1 ). PCR was performed with Quick-Load Taq 2x Master-Mix (New England Biolabs). The PCR product was digested with Nde I/ Xho I and ligated into pET22b+ cut with the same restriction enzymes. Plasmid pPJ8 (pKSM/SufI-ss-ex) was generated by inverse PCR as described for plasmid pPJ6 ( [29] ) using the primers SufI ss ex. for and SufI ss ex. rev and pKSMSufI-RR [23] as template. To construct plasmid pPJ9 (pASK-IBA33plus/SufI), the SufI-encoding DNA sequence was amplified via PCR using Pfu Polymerase (Fermentas), pKSMSufI-RR [23] as template and the primers SufI IBA3 for and SufI IBA3 rev. The PCR fragment and the recipient vector pASK-IBA33plus were digested with Bsa I and ligated. To construct plasmid pPJ10 (pBAD33/TatC), the TatC-encoding DNA sequence was amplified via PCR using Pfu Polymerase, plasmid p8737 as template [55] and the primers 5′-SacI TatC and 3′-BglII TatC. The PCR fragment and the recipient vector pBAD33 were digested with Sac I and Bgl II and ligated following dephosphorylation of the vector by antarctic phosphatase (New England Biolabs). To add a Shine-Dalgarno sequence upstream of TatC, the resulting plasmid was linearized with Sac I, followed again by dephosporylation. It was then incubated for 5 min at room temperature with the phosporylated oligos P-SacI pBAD for and P-SacI pBAD rev that encode the Shine-Dalgarno sequence present in pET22b+ and finally re-ligated. Owing to the cloning strategy, two additional amino acids were added to the C-terminus of TatC. Plasmid p8737-tatAC was constructed to generate a tatAC expression vector with a tatA upstream region that is similar to the tatABCD expression vector p8737 using a ‘crossover’-PCR method. First the tatA upstream region from p8737 was amplified by using the forward primer LacI_int_vorne_for and the reverse Primer Co_p8737_AC_rev with p8737 serving as template. Next, the tatAC operon was amplified by using the forward primer Co_AC_p8737_for, which has a 5′-extension that is complementary to the 3′-end of the first PCR product, and the reverse primer TatC_Ende_NdeI_rev with pHSG-TatAC [40] as template. Both fragments were purified and used as a template in a crossover PCR using primers LacI_int_vorne_for and TatC_Ende_NdeI_rev. The obtained PCR fragment was digested with XbaI and Nde I and ligated into the Xba I/ Nde I digested p8737 plasmid backbone, resulting in plasmid p8737-tatAC. All PCR reactions were carried out using the Expand High Fidelity PCR system (Roche). Plasmids pKSMSufI-RR encoding SufI [23] , pET28aTorA-PhoA and pET28aTorA-PhoAΔSP encoding TorA-PhoA and a non-cleavable variant of it [27] , pPJ1 encoding TorA-MalE335 lacking the 35 C-terminal residues of MalE [52] , pPJ2 encoding TorA(KK)-MalE335 ( [29] ), pPJ3 encoding TorA-mCherry [52] , pPJ4 encoding SufI [29] , pPJ5 encoding TorA(KK)-mCherry [52] , pPJ6 ( [29] ) encoding TorA-SufIΔLinker, which is a linker-less version of TorA-SufI encoded by pPJ4, pTF1 encoding AmiC [29] , p8737 containing an T7-dependent tatABCD operon [55] , and pFAT588 encoding a hexa-histidine-tagged version of TatC [56] have been described previously. In vitro reactions S-135 cell extracts were obtained from E. coli strains SL119 ( [57] ) and Top10 (Invitrogen). Cells were grown and S-135 cell extracts were prepared as described [43] . Coupled transcription/translation of the different precursor proteins from plasmid DNAs was performed as described [43] . Tat-dependent translocation of TorA-PhoA requires oxidizing conditions [27] . Those were established by the addition of 5 mM oxidized glutathione (GSSG) at the start of synthesis. Membrane vesicles were added 10 min after starting the synthesis reaction and incubated for 25 min at 37 °C. For assaying translocation of precursors into INV, 15 μl of each reaction were treated with 15 μl 10% (w/v) trichloroacetic acid (TCA) and 30 μl were incubated with PK according to Moser et al. [43] Where appropriate, CCCP was added at 0.1 mM final concentration together with INV. For sodium carbonate extraction, a 50 μl reaction was treated with 50 μl freshly prepared, ice- cold 0.4 M Na 2 CO 3 . After 30 min at 4 °C, samples were centrifuged for 30 min at 70,000 r.p.m. in a Beckman TLA100 ultracentrifuge (Beckman-Coulter) using a TLA 100.3 rotor. Afterwards supernatants were precipitated with 100 μl 10% (w/v) TCA and resuspended in SDS–PAGE loading buffer. The pellets were solubilized directly in 30 μl SDS-PAGE loading buffer. Preparation of membrane vesicles INV were prepared as described previously [43] from E. coli strain BL21(DE3)ΔTat (B. Ize and T. Palmer, personal communication) transformed with plasmid p8737 (Tat + -INV), p8737-tatAC (TatAC-INV) and pFAT588 (TatC-INV). Expression of tat genes was induced with 1 mM isopropyl β- D -thiogalactopyranoside during the growth of cells from an optical density (OD) at 600 nm of 0.5 up to 2.0. In vivo labelling of Tat precursors Strains BL21(DE3), BL21(DE3)ΔTat (see above) and BL21(DE3)ΔTat containing plasmid pPJ10 (TatC) were transformed with plasmids pPJ9, pPJ3 and pPJ7 each. M63 minimal media supplemented with 10 mg l −1 thiamine hydrochloride, 100 μM each of 18 amino acids except methionine and cysteine, and the appropriate antibiotics were inoculated with overnight cultures of the respective strains to give an OD at 600 nm of 0.1. After growth at 37 °C to an OD 600 of 0.25–0.3, cells-harbouring plasmid pPJ10 (TatC) were induced with 0.1% arabinose. At an OD 600 of 0.5–0.6, 250 μl of cell cultures expressing pSufI, and 500 μl of cell cultures expressing TorA-mCherry and pNapG were each transferred to microfuge tubes and placed in an Eppendorf Thermomixer set at 37 °C. Cells were pulsed with 4 μl ml −1 35 [S]-methionine/cysteine (11–15 μCi/μl) and simultaneously treated with either 200 ng ml −1 anhydrotetracycline dissolved in dimethylsulphoxide to induce synthesis of pSufI from pPJ9 or with at least 1 mM β- D -thiogalactopyranoside to induce synthesis of TorA-mCherry from plasmid pPJ3 and pNapG from plasmid pPJ7, respectively. After 5 min of pulse time in the case of pSufI and after 15 min in the case of TorA-mCherry and pNapG, cells were chased with non-labelled methionine and cysteine (500 μg ml −1 final concentration) for 60 min. Reactions were stopped by the addition of 5% TCA (final concentration) and incubation on ice for 30 min. TCA precipitates were collected, dissolved in dithiothreitol-free SDS–PAGE loading buffer, treated with 8 M urea and applied to Ni-Sepharose as described [58] in order to isolate His-tagged SufI, TorA-mCherry and NapG species. Miscellaneous For western blotting, 4 μl INV (A 280 ~40 μ ml −1 ) were each dissolved in 96 μl SDS–PAGE loading buffer. Of this solution, 5 μl were used for SDS–PAGE and western transfer, when blots were decorated with anti-TatA antibodies, and 20 μl when using anti-TatB and anti-TatC antibodies. Polyclonal antibodies against TatA, TatB and TatC were raised in rabbits as described [23] , [55] . The second antibody was goat anti-rabbit IgG coupled to alkaline phosphatase (Sigma). Detection was performed using NBT/BCIP Stock Solution (Roche) following the manufacturer’s instructions. SDS–electrophoresis using 10% polyacrylamide gels was performed as described previously [43] . How to cite this article : Fröbel, J. et al. Transmembrane insertion of twin-arginine signal peptides is driven by TatC and regulated by TatB. Nat. Commun. 3:1311 doi: 10.1038/ncomms2308 (2012).